Coupling artificial molecular spin states by photon-assisted tunnelling Artificial molecules containing just one or two electrons provide a powerful platform for studies of orbital and spin quantum dynamics in nanoscale devices. A well-known example of these dynamics is tunnelling of electrons between two coupled quantum dots triggered by microwave irradiation. So far, these tunnelling processes have been treated as electric-dipole-allowed spin-conserving events. Here we report that microwaves can also excite tunnelling transitions between states with different spin. We show that the dominant mechanism responsible for violation of spin conservation is the spin–orbit interaction. These transitions make it possible to perform detailed microwave spectroscopy of the molecular spin states of an artificial hydrogen molecule and open up the possibility of realizing full quantum control of a two-spin system through microwave excitation. In recent years, artificial molecules in mesoscopic systems have drawn much attention owing to a fundamental interest in their quantum properties and their potential for quantum information applications. Arguably, the most flexible and tunable artificial molecule consists of coupled semiconductor quantum dots that are defined in a two-dimensional electron gas using a set of patterned electrostatic depletion gates. Electron spins in such quantum dots exhibit coherence times up to 200 μs (ref. 1 ), about 10 4 –10 6 times longer than the relevant quantum gate operations [2] , [3] , [4] , making them attractive quantum bit (qubit) systems. [5] The molecular orbital structure of these artificial quantum objects can be probed spectroscopically by microwave modulation of the voltage applied to one of the gates that define the dots [6] . In this way, the delocalized nature of the electronic eigenstates of an artificial hydrogen-like molecule was observed [7] , [8] . More recently, electrical microwave excitation was used for spectroscopy of single spins [9] , [10] , [11] and coherent single-spin control [9] , [11] , through electric-dipole spin resonance. Here we perform microwave spectroscopy [7] , [8] , [12] on molecular spin states in an artificial hydrogen molecule formed by a double quantum dot (DD) which contains exactly two electrons. In contrast to all previous photon-assisted tunnelling (PAT) experiments, we observe not only the usual spin-conserving tunnel transitions, but also transitions between molecular states with different spin quantum numbers. We discuss several possible mechanisms and conclude from our analysis that these transitions become allowed predominantly through spin–orbit (SO) interaction. The possibility to excite spin-flip tunnelling transitions lifts existing restrictions in our thinking about quantum control and detection of spins in quantum dots, and allows universal control of spin qubits without gate-voltage pulses. 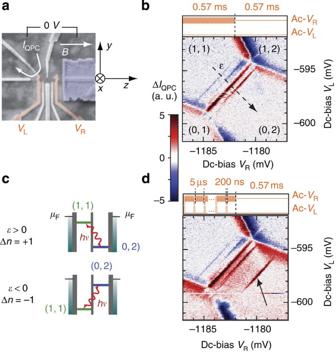Figure 1: Photon-assisted tunnelling in a 2-electron double quantum dot. (a) Scanning-electron micrograph top view of the double-dot gate structure with Co micromagnet (blue). The voltages applied to the leftVLand rightVRside gates (red) control the detuningɛof the double-dot potential. The double-dot charge state is read out by means of the currentIQPCrunning through a nearby quantum point contact (white arrow). (b) Charge stability diagram around the 2-electron regime atB=1.5 T. (nL,nR) indicate the absolute numbers of electrons in the left and right dot, respectively. During measurements, 11 GHz microwaves with 880 Hz on–off modulation are applied to the right side gate. The top panel displays schematically one cycle of the ac signal applied to the right side gate. Along the detuning axis (dashed arrow) PAT-lines are observed. (c) In the conventional picture of PAT, the first sidebands seen inbshould appear when the detuning of the (0,2) and (1,1) states matches the photon energy, and interdot tunnelling is induced. Further sidebands are then interpreted as multi-photon transitions.μFis the chemical potential of the left and right electron reservoir. (d) Same as inb, but the microwaves are interrupted every 5 μs by a 200 ns,Pɛ=2 mV detuning pulse applied to the left and right side gates (see the schematic in the top panel). The pulses generate a reference line (black arrow) due to mixing at theST+anti-crossing. Device and excitation protocol Figure 1a displays a scanning electron micrograph of a sample similar to that used in the experiments. It shows the metal gate pattern that electrostatically defines a DD and a quantum point contact (QPC) within a GaAs/(Al,Ga)As two-dimensional electron gas. An on-chip Co micro-magnet (μ magnet) indicated in blue in Figure 1a generates an inhomogeneous magnetic field across the DD, which adds to the homogeneous external in-plane magnetic field B (Methods), but is not needed for the molecular spin spectroscopy. The sample was mounted in a dilution refrigerator equipped with high-frequency lines. The gate voltages are set so that the DD can be considered as a closed system (the interdot tunnelling rates are 10 4 times larger than the dot-to-lead tunnelling rates), and the tilt of the DD potential is tuned by the dc-voltages V L and V R , applied to the left and right side gates. Working near the turn-on of the first conductance plateau, the current through the QPC, I QPC , depends upon the local charge configuration and provides a sensitive meter for the absolute number of electrons ( n L , n R ) in the left and right dot, respectively [13] , [14] . Figure 1: Photon-assisted tunnelling in a 2-electron double quantum dot. ( a ) Scanning-electron micrograph top view of the double-dot gate structure with Co micromagnet (blue). The voltages applied to the left V L and right V R side gates (red) control the detuning ɛ of the double-dot potential. The double-dot charge state is read out by means of the current I QPC running through a nearby quantum point contact (white arrow). ( b ) Charge stability diagram around the 2-electron regime at B =1.5 T. ( n L , n R ) indicate the absolute numbers of electrons in the left and right dot, respectively. During measurements, 11 GHz microwaves with 880 Hz on–off modulation are applied to the right side gate. The top panel displays schematically one cycle of the ac signal applied to the right side gate. Along the detuning axis (dashed arrow) PAT-lines are observed. ( c ) In the conventional picture of PAT, the first sidebands seen in b should appear when the detuning of the (0,2) and (1,1) states matches the photon energy, and interdot tunnelling is induced. Further sidebands are then interpreted as multi-photon transitions. μ F is the chemical potential of the left and right electron reservoir. ( d ) Same as in b , but the microwaves are interrupted every 5 μs by a 200 ns, P ɛ =2 mV detuning pulse applied to the left and right side gates (see the schematic in the top panel). The pulses generate a reference line (black arrow) due to mixing at the ST + anti-crossing. Full size image First, we excite the DD as indicated in the top panel of Figure 1b , by adding to V R continuous-wave microwave excitation at fixed frequency ν =11 GHz. When the photon energy of the microwaves matches the energy splitting between the ground state and a state with a different charge configuration, a new steady-state charge configuration results, which is visible as a change in the QPC current, Δ I QPC . The excitation is on–off modulated at 880 Hz and lock-in detection of Δ I QPC reveals the microwave-induced change of the charge configuration (see Methods for further experimental details). The lower panel of Figure 1b shows Δ I QPC as a function of V L and V R near the (1,1) to (0,2) boundary of the charge stability diagram. Sharp red (blue) lines indicate microwave-induced tunnelling of an electron from the right to the left dot (left to right), labelled as Δ n =+1 (Δ n =−1), respectively ( Fig. 1c ). Sidebands can result from multi-photon absorption. At the boundaries with the (0,1) and (1,2) charge states, no energy quantization is observed, because, here, electrons tunnel to and from the electron-state continuum of the leads. At first sight, the observations in Figure 1b thus appear to be well explained by the usual spin-conserving PAT processes. Surprisingly, the position in gate voltage of the resonant lines exhibits a striking dependence on the in-plane magnetic field, B . 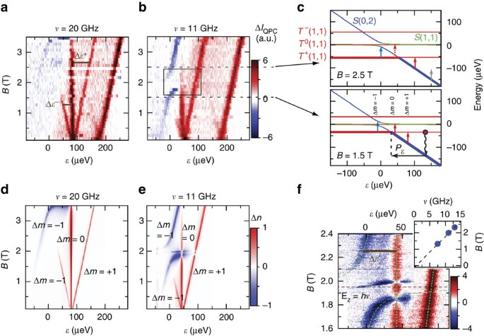Figure 2: Photon-assisted-tunnelling spectra and simulations. (a,b) Microwave-induced change of the QPC current ΔIQPCas a function of the double-dot detuningɛand the external magnetic fieldBfor 20 GHz (a) and 11 GHz (b) frequency, respectively. Singlet–triplet mixing due to 2-mV detuning pulses generates a reference signal that is used to calibrate the detuning axis (see lower panel inFig. 2f). (c) Eigenenergies versus double-dot detuningɛof the two-electron spin states in the (1,1) and (0,1) charge regime for two external magnetic fieldsB=2.5 T (upper panel) andB=1.5 T (lower panel), respectively.S(0,2),S(1,1) andT(1,1) character of the eigenstates is indicated by blue, green and red colour, respectively. The molecular spin ground state is indicated by thick lines. The vertical arrows indicate PAT transitions for a constant microwave frequency involving spin flips. The transition indicated by a dashed arrow is suppressed, because the initial state lies above the ground state. The red circle in the lower panel indicates the detuning position of the reference signal, that is generated by a detuning pulse with amplitudePɛto theST+anti-crossing. (d,e) Simulated PAT spectra for 20 GHz (a) and 11 GHz (b) frequency, respectively. The colour indicates the change of the population of the steady-state charge state Δnas would be observed in an on–off lock-in detection. A finite temperature of 100 mK and spontaneous relaxation through the phonon bath are taken into account. (f)IQPCscanned with higher resolution in the anti-crossing region (black rectangle inFig. 2b) at 11 GHz excitation. The green dashed lines indicate the expected detuning positions of the PAT transitions. The horizontal black dashed line indicates the magnetic field, at which the electron spin resonance condition is fulfilledEz=gμB(B+b0)=hv. The graph is concatenated from two scans that overlap at 1.9 T. The inset displays three magnetic fields (blue dots), at which the centre of the horizontal blue triplet resonance line is observed, as a function of the microwave frequency ν. The dashed black line gives the expected position of the triplet resonance. This is clearly seen in Figure 2a,b , which display the measured PAT spectrum along the DD detuning ɛ axis (dashed black arrow in Fig. 1b ) as a function of B for 20 and 11 GHz excitation, respectively. Figure 2: Photon-assisted-tunnelling spectra and simulations. ( a , b ) Microwave-induced change of the QPC current Δ I QPC as a function of the double-dot detuning ɛ and the external magnetic field B for 20 GHz ( a ) and 11 GHz ( b ) frequency, respectively. Singlet–triplet mixing due to 2-mV detuning pulses generates a reference signal that is used to calibrate the detuning axis (see lower panel in Fig. 2f ). ( c ) Eigenenergies versus double-dot detuning ɛ of the two-electron spin states in the (1,1) and (0,1) charge regime for two external magnetic fields B =2.5 T (upper panel) and B =1.5 T (lower panel), respectively. S (0,2), S (1,1) and T (1,1) character of the eigenstates is indicated by blue, green and red colour, respectively. The molecular spin ground state is indicated by thick lines. The vertical arrows indicate PAT transitions for a constant microwave frequency involving spin flips. The transition indicated by a dashed arrow is suppressed, because the initial state lies above the ground state. The red circle in the lower panel indicates the detuning position of the reference signal, that is generated by a detuning pulse with amplitude P ɛ to the ST + anti-crossing. ( d,e ) Simulated PAT spectra for 20 GHz ( a ) and 11 GHz ( b ) frequency, respectively. The colour indicates the change of the population of the steady-state charge state Δ n as would be observed in an on–off lock-in detection. A finite temperature of 100 mK and spontaneous relaxation through the phonon bath are taken into account. ( f ) I QPC scanned with higher resolution in the anti-crossing region (black rectangle in Fig. 2b ) at 11 GHz excitation. The green dashed lines indicate the expected detuning positions of the PAT transitions. The horizontal black dashed line indicates the magnetic field, at which the electron spin resonance condition is fulfilled E z = gμ B (B+ b 0 )= hv . The graph is concatenated from two scans that overlap at 1.9 T. The inset displays three magnetic fields (blue dots), at which the centre of the horizontal blue triplet resonance line is observed, as a function of the microwave frequency ν. The dashed black line gives the expected position of the triplet resonance. Full size image As the gate constitutes an open-ended termination of the transmission line, the excitation produces negligible AC magnetic fields at the DD (estimated in Methods), and is, therefore, expected to give rise to only electric-dipole-allowed spin-conserving transitions, with no B dependence. Furthermore, there is a pronounced asymmetry between the position of the red and blue PAT lines. In these figures, the detuning axis was calibrated for all magnetic fields by introducing a reference line ( Fig. 1d , black arrow) that facilitates interpretation of the spectra despite residual orbital effects of the magnetic field. This line was produced by interspersing the microwaves every 5 μs with 200 ns gate-voltage pulses along the detuning axis (see the top panel in Fig. 1d ), leading to singlet–triplet mixing as described in ref. 2 . The short gate-voltage pulses do not noticeably alter the position of the PAT lines (compare Fig. 1b,d ). The reference peaks visible at around ɛ =200 μeV in Figure 2a,b were aligned by shifting all data points at a given B by the same amount in detuning (see Supplementary Note 1 'Calibration of the detuning axis' for the full details of this post-processing step and Supplementary Fig. S1a–d for the corresponding spectra). Interpretation of the photon-assisted tunnelling spectra The complexity of the PAT spectra shown in Figure 2a,b can be understood in detail, if we allow for non-spin conserving transitions. The two diagrams in Figure 2c show the energies of all relevant DD-states (four (1,1)-states and one singlet S (0,2)-state) as a function of ɛ for two different (fixed) magnetic fields, that is, the spectrum of the DD along the two horizontal dotted lines in Figure 2b [15] . Note that the only difference between the two diagrams is the splitting between the three triplet T (1,1)-states. First, we explain the resonances observed along the upper dotted line in Figure 2b ( B =2.5 T). In the corresponding (upper) diagram in Figure 2c , we plot the ground state energy for all ɛ with a thick line. If the microwave excitation is off-resonance with all transitions, the system will be in this ground state. For instance, at ɛ =150 μeV, there is no state available 11 GHz above the S (0,2) ground state (grey arrow) and the system stays in S (0,2). However, when decreasing the detuning, at some point T + (1,1) becomes energetically accessible (red arrow) and, because we allow for non-spin-conserving transitions, is populated owing to the microwave excitation. For this PAT transition, the spin projection on the quantization axis is changed by Δ m =+1. The resulting change of steady-state charge population (increased population of (1,1), or Δ I QPC >0) is detected by the QPC and yields the red peak in Figure 2b . Decreasing ɛ further, there are two more resonances detectable: (i) the S (0,2)− S (1,1) transition (dotted red arrow, Δ m =0), although the signal will be weakened owing to the fact that S (0,2) is not unambiguously the ground state anymore. Note that a transition S (0,2)− T 0 (1,1) could appear in nearly the same detuning position, as will be discussed below. (ii) the T + (1,1)- S transition (blue arrow), where S stands for the hybridized S (0,2)− S (1,1) singlet, results in a negative (blue, Δ I QPC <0, Δ m =−1) signal from the charge detector as the ground state is now (1,1) and the excited state is partly (0,2). We see that this simple analysis explains both the positions and the signs of the resonances observed in the data. A similar analysis can be made for other magnetic fields. For instance, for the spectrum plotted in the lower diagram of Figure 2c, we find two resonances with Δ I QPC >0 (red arrows), and one with Δ I QPC <0 (blue arrow). Note that the `blue' transition now connects the ground state to the other branch of the hybridized S compared to the high magnetic field case. Indeed, the singlet anti-crossing is directly probed, resulting in the two blue curved lines observed in the data around ɛ =0 ( Fig. 2b ). The fading out of the blue signal at low fields can be understood from pumping into the metastable state S (1,1): the microwaves excite the system from T + (1,1) to S (0,2), from where it relaxes quickly to S (1,1). However, relaxation from S (1,1) back to the ground state is slow because of the small energy difference of this transition and the small phonon density of states at low energies [14] , [16] . This pumping weakens the detector signal, as S (1,1) has the same charge configuration as the ground state. To verify this interpretation, we calculate in Figure 2d,e the position and intensity of the spectral lines at fixed microwave frequency, on the basis of the energy level diagram of Figure 2c . In the simulations, all single-photon transitions between the ground state and the excited states are allowed by including a matrix element | T ± (1,1)〉〈 S (0,2)| (Methods). The input parameters for the calculation of the resonant positions are the interdot S (1,1) to S (0,2) tunnel coupling t s , the absolute electron g -factor | g| , a magnetic-field contribution b 0 from the μ magnet parallel to B as well as a magnetic field gradient between the dots (in Fig. 3 , we show how t s , | g| and b 0 can be extracted from the experimental spectra). The colour scale represents the calculated steady-state Δ n that results from microwave excitation, orbital hybridization, and phonon absorption and emission at 100 mK. All the PAT transitions visible in the simulation also appear in the experiment, with excellent agreement in both the position and relative intensity of the spectral lines. Especially, the vanishing signal due to spin pumping is also predicted by the simulations that include phonon relaxation. Surprising at first glance, the intensities of the spin-flip lines Δ m =±1 and the spin-conserved line Δ m =0 are about the same, which holds true for both simulation and measurement, although Δ m =0 has a larger matrix element. This is because the same matrix elements enter the spontaneous phonon-mediated relaxation rates, resulting in similar steady-state populations for the two transitions. 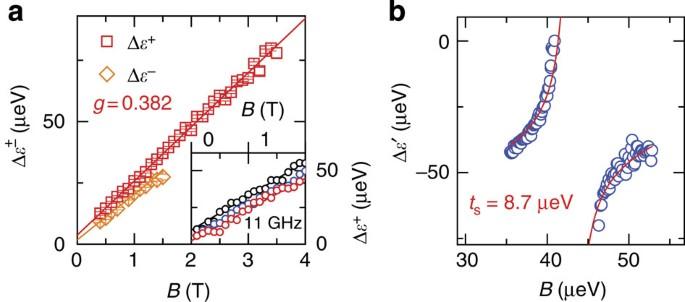Figure 3: Analysis of the photon-assisted-tunnelling spectra. (a) The detuning difference Δɛbetween the spin-conserving line Δm=0 and the Δm=±1 line is plotted as a function of the external magnetic fieldBat 20 GHz (seeFig. 2a), to fit the absolute effective electron g-factorgfrom the slopes of the linear fits (solid lines). inset, Δɛfor the Δm=+1 line at 11 GHz for different tunnel couplings. The offset of the curves increases with increasingts(red to black circles) whilegremains constant. (b) Δɛbetween the Δm=0 line and the Δm=−1 (1,1) to (0,2) transition fromFigure 2c. The fit of the anti-crossing (red line) allows for a precise determination ofts. Figure 3: Analysis of the photon-assisted-tunnelling spectra. ( a ) The detuning difference Δ ɛ between the spin-conserving line Δ m =0 and the Δ m =±1 line is plotted as a function of the external magnetic field B at 20 GHz (see Fig. 2a ), to fit the absolute effective electron g-factor g from the slopes of the linear fits (solid lines). inset, Δ ɛ for the Δ m= +1 line at 11 GHz for different tunnel couplings. The offset of the curves increases with increasing t s (red to black circles) while g remains constant. ( b ) Δ ɛ between the Δ m= 0 line and the Δ m= −1 (1,1) to (0,2) transition from Figure 2c . The fit of the anti-crossing (red line) allows for a precise determination of t s . Full size image When we zoom in on the boxed region of Figure 2b , we see an extra horizontal blue feature at B ≈2 T ( Fig. 2f ) that also appears in the calculated spectra of Figure 2e . This feature is due to a triplet resonance from T + (1,1) to T 0 (1,1) that becomes detectable by relaxation into the meta-stable S (0,2) state. In the detuning range where this line appears, the S (0,2) state lies energetically only slightly above the T + (1,1) state, so relaxation back to the T + (1,1) ground state is suppressed, again by the small phonon density of states at low energies (see Supplementary Fig. S2a for a schematic energy diagram). The triplet resonance is expected to appear at E z = gμ B ( B + b 0 )= hν , where h is Planck's constant and μ B the Bohr magneton. The inset of Figure 2f shows the magnetic fields corresponding to the centre of the measured triplet resonance line for three excitation frequencies (see Supplementary Note 2 'Triplet spin resonance' for details and Supplementary Fig. S2b,c for extra spectra taken at different microwave frequencies), which are in good agreement with the expected positions (black dashed lines in Fig. 2f ) based on the values | g | and b 0 determined in the next section from other features of the PAT spectra. Surprisingly, the measured triplet resonance exhibits a finite slope in the B ( ɛ ) spectra. A longitudinal magnetic field gradient ΔB || gives rise to such a detuning dependence, but the ΔB || required in our simulations to reproduce the observed slope is ΔB || ≳ 80 mT per 50 nm, an order of magnitude larger than the gradient we calculate for the μ magnet. The magnitude of the slope remains a puzzle. Extracting artificial molecule parameters We now show how | g |, t s and b 0 , the parameters used for all simulations, can be extracted independently from the experimental spin-flip PAT spectra. For this analysis, we only use the relative distance Δ ɛ between PAT lines at fixed magnetic field, to be independent from the calibration of the detuning axis by means of the reference line. Figure 3a shows Δ ɛ ± as a function of B using the 20 GHz data. Δ ɛ ± is defined as the difference in detuning between the red Δ m =±1 and Δ m =0 PAT lines as plotted in Figure 2a . For a fixed ν , both Δ ɛ ± increase linearly with the Zeeman energy and therefore allow fitting of |g|. (Note that for Δ ɛ + the linearity is only exact for sufficiently large B , at which the singlet anti-crossing does not affect the detuning position of the S(0,2) to T + (1,1) transition. A least-squares fit to the Δ ɛ + data gives | g |=0.382±0.004 ( Fig. 3a ). From the linear behaviour of Δ ɛ + , we also deduce that there is most likely negligible dynamic nuclear polarization in the experiment. Knowing | g | precisely, we make use of the blue anti-crossing in Figure 2b,f to determine t s (and b 0 ). Figure 3b shows the difference in detuning Δ ɛ ′ between the blue Δ m =−1 and the red Δ m =0 lines in Figure 2f . Assuming the Δ m =0 line corresponds to the S (0,2)- S (1,1) transition (as shown below), then where the first term is the detuning position of the T + (1,1)- S transition and the second the one of the S (0,2)− S (1,1) transition. The best fits are obtained with t s =8.7±0.1 μeV and b 0 =109±16 mT. This value for b 0 matches our simulations of the stray field of the μ magnet at the DD location very well (see Methods ). An important question left open so far is whether the red Δ m =0 line involves predominantly transitions from S (0,2) to S (1,1) or to T 0 (1,1). The transition to S (1,1) does not require a change in the (total) spin and is thus expected to be excited more strongly than that to T 0 (1,1). However, relaxation from S (1,1) back to S (0,2) will be stronger as well, so it is not obvious what steady-state populations will result in either case. Furthermore, given the small energy difference between S (1,1) and T 0 (1,1), the two transitions are not resolved in Figure 2 . Figure 3a helps to answer this question: The observation that Δ ɛ + >Δ ɛ − indicates that the Δ m =0 line originates from the transition to S (1,1) and not to T 0 (1,1). For the former we expect Δ ɛ ± = E z ± J , with the exchange energy, whereas the latter would result in Δ ɛ + ≲ Δ ɛ − (in both scenarios, b 0 causes an extra fixed offset in both Δ ɛ ± , but it does not contribute to their difference; for transitions to both S (1,1) and T 0 (1,1), we plotted the expected Δ ɛ ± ( B ) dependence for our DD parameters in the Supplementary Fig. 3a ). This interpretation is consistent with the increase of Δ ɛ + with larger interdot tunnel coupling, hence larger J ( Fig. 3a inset; the slopes are not affected). In Supplementary Note 3 'The Δ m =0 PAT transition', we give more arguments for our interpretation by analysing quantitatively the intercept Δ ɛ + ( B =0 T) for various microwave frequencies, as plotted in Supplementary Figure S3b . So far only single-photon processes were considered, but at higher microwave power, also multi-photon lines emerge ( Fig. 4a ), mostly for the S (0,2)− S (1,1) transition (green dashed lines in Fig. 4a ). Like the single-photon S (0,2)− S (1,1) line, their position in detuning is B -independent. 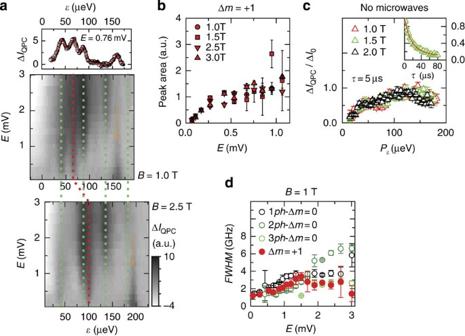Figure 4: Power-dependence of the photon-assisted tunnelling spectra and spontaneous relaxation. (a) ΔIQPCas a function of the double-dot detuningɛand the microwave amplitudeEfor 11 GHz andB=1.0 T (middle panel) andB=2.5 T (lower panel). The excitation scheme fromFigure 1dis employed with reference pulse amplitudePɛ=1.5 mV. The green (red) dashed lines mark the multi-photon Δm=0 (Δm=+1) PAT transitions. The reference signal stemming from the pulse is marked by orange arrows. The voltage amplitudeEis measured at the end of the coaxial lines at room temperature. The uppermost panel displays a linecut measured at 1 T. The red line is a least-squares fit by a sum of four lorentzian peaks to the data. (b) The fitted Lorentzian peak area of the Δm=+1 line fromais plotted as a function of microwave amplitudeEand magnetic fieldB. (c) Normalized QPC current averaged overτ=5 μs immediately after full mixing at theST+anticrossing for various magnetic fields at zero microwave power. The spontaneous spin relaxation after mixing is measured at a distancePɛto theST+mixing point (see scheme inFig. 2c). The dependence on the averaged time intervalτis displayed in the inset forB=1.5 T andPɛ=2 mV together with a least-squares fit (red solid line). (d) The fitted Lorentzian linewidth at half maximum (FWHM) of the Δm=+1 and the lines Δm=0 fromais plotted as a function of microwave amplitudeEforB=1 T. The error bars inb,dare determined from the Lorentzian least-squares fit (see the upper panel ofFig. 4a). Figure 4: Power-dependence of the photon-assisted tunnelling spectra and spontaneous relaxation. ( a ) Δ I QPC as a function of the double-dot detuning ɛ and the microwave amplitude E for 11 GHz and B =1.0 T (middle panel) and B =2.5 T (lower panel). The excitation scheme from Figure 1d is employed with reference pulse amplitude P ɛ =1.5 mV. The green (red) dashed lines mark the multi-photon Δ m= 0 (Δ m= +1) PAT transitions. The reference signal stemming from the pulse is marked by orange arrows. The voltage amplitude E is measured at the end of the coaxial lines at room temperature. The uppermost panel displays a linecut measured at 1 T. The red line is a least-squares fit by a sum of four lorentzian peaks to the data. ( b ) The fitted Lorentzian peak area of the Δ m= +1 line from a is plotted as a function of microwave amplitude E and magnetic field B . ( c ) Normalized QPC current averaged over τ =5 μs immediately after full mixing at the ST + anticrossing for various magnetic fields at zero microwave power. The spontaneous spin relaxation after mixing is measured at a distance P ɛ to the ST + mixing point (see scheme in Fig. 2c ). The dependence on the averaged time interval τ is displayed in the inset for B =1.5 T and P ɛ =2 mV together with a least-squares fit (red solid line). ( d ) The fitted Lorentzian linewidth at half maximum ( FWHM ) of the Δ m =+1 and the lines Δ m =0 from a is plotted as a function of microwave amplitude E for B =1 T. The error bars in b , d are determined from the Lorentzian least-squares fit (see the upper panel of Fig. 4a ). Full size image Having shown the power of spin-flip PAT for detailed molecular spin spectroscopy, we now discuss the mechanisms responsible for this process as confirmed by our simulations. As a first possibility, the transitions from S (0,2) to the triplet (1,1) states can take place through a virtual process involving S (1,1): the state S (0,2) is coupled to S (1,1) by the interdot tunnel coupling, and an (effective) magnetic field gradient across the DD couples the spin part of all the (1,1) states to each other [14] , [17] . Here has a contribution from the effective nuclear field and from the μ magnet. The transition matrix element from S (0,2) to T ± (1,1) is , assuming E z = J . In the following, we use the B -dependence of this process as a fingerprint and focus on the red Δ m =+1 line in Figure 2a,b , as we can follow it over the entire magnetic field range. The intensity of this line is constant in B , and even if the microwave amplitude E is varied, we observe no B -dependence in the area under this peak ( Fig. 4b ). This does not in itself provide evidence that the transition rate is magnetic field independent. As stated above, the observed PAT lines reflect the steady-state change in the charge configuration resulting from stimulated photon emission and absorption, and spontaneous relaxation. A field-independent steady state could thus be reached from a field dependence of relaxation and excitation that cancel each other. We therefore verify that the spontaneous relaxation rate is field-independent as well. The measurement of the spontaneous relaxation rate is done as follows: Starting from S (0,2), we populate the T + (1,1) by 50% through a 200-ns detuning pulse [18] with amplitude P ɛ in the absence of microwaves, and monitor the decay back to S (0,2). The relaxation rate Γ s can be extracted from the time-averaged lock-in signal where τ is the time spent in Pauli blockade between the pulses. Δ I 0 = I QPC (0), which is independent from B , is extracted from the fit in the inset of Figure 4c . To cover various values of the detuning and the magnetic field, we next fix τ =5 μs and record Δ I QPC as a function of P ɛ for three different magnetic fields. We observe that Δ I QPC (5 μs) and thus Γ s are essentially independent of B ( Fig. 4c ). This holds true for all P ɛ and hence for all T + (1,1)- S (0,2) energy splittings. Note that regardless of B , this energy splitting is given by P ɛ alone. This reflects exactly the situation in the PAT experiment, for which the microwave frequency alone sets the energy splitting and, thus, also the required phonon energy for the spontaneous relaxation process. The field-independence of relaxation suggests that the coupling mechanism is magnetic field independent, and, thus, virtual processes involving S (1,1) do not give a strong contribution to the transition rates. More recently, two mechanisms were considered that provide a direct, B -independent matrix element between S (0,2) and the (1,1) triplet states: (i) the hyperfine contact Hamiltonian is of the form Thus, nuclear spins, , in the barrier regions, where the left-dot and right-dot orbitals overlap, can flip-flop with the electron spin, , simultaneously with charge tunnelling [19] . (ii) The SO Hamiltonian is of the form p x,y S x,y and can directly couple states that differ in both orbital and spin [20] , [21] . (When the orbital part of the initial and final state are the same, the SO Hamiltonian does not provide a direct matrix element, and the transition rate becomes B -dependent. [9] , [22] , [23] , [24] , [25] ) The ratio of the SO-mediated rate and the hyperfine mediated rate can be estimated as , which is a few thousand in the experiment (see Supplementary Note 4 'Spin flip tunnelling mechanism' for the derivation). Here Δ is the single-dot level spacing, N the number of nuclei in contact with one dot, A the hyperfine coupling strength, a the interdot distance and λ so the spin–orbit length. We, therefore, believe that SO interaction is the dominant spin-flip mechanism for the observed PAT transitions. The presence of a magnetic-field-independent matrix element between S (0,2) and the (1,1) triplets is confirmed by the observation that the intensity of the reference signal shows no field dependence. Finally, we extract from Figure 4a the fitted linewidth as a function of driving power ( Fig. 4d ). For small E , we find a width ≳ 1 GHz, similar to that observed earlier for spin-conserving PAT processes [7] . For stronger driving, both the Δ m =0 and the Δ m =+1 lines are further broadened, up to E ∼ 1.5 mV. If these lines were power broadened, their width would imply transition rates in excess of 1 GHz. However, we do not believe that this is the case, because, in measurements with short microwave bursts, the populations saturated only on a long (10-μs) timescale (data not shown). Presumably, charge or gate-voltage noise is responsible for the broadening instead. We have shown that in our DD system, all (1,1) spin states have at least weakly allowed electric-dipole transitions to S (0,2). In materials with high SO interaction like InAs, the effect of the non-spin conserving PAT will be even stronger. In materials with weak SO interaction, a strong gradient magnetic field can be used to facilitate spin-flip tunnelling transitions. In all cases, all (1,1) to S (0,2) transitions can be driven. This opens up the possibility of realizing full quantum control of the two spins in the (1,1) manifold through off-resonant (microwave) -stimulated Raman transitions through the excited S (0,2) state, at small negative detuning and in the presence of a finite Δ B || . Furthermore, we find from our analysis that the vicinity in energy of the S (0,2) state also allows direct (single-frequency) transitions to be induced between any two–spin states within the (1,1) subspace. Direct and stimulated Raman transitions are governed by the same matrix elements (see Methods ). The calculated Rabi frequencies Ω ij for the direct transitions are shown in Table 1 . For each pair of states, the dephasing rate γ ij from phonon decay and co-tunnelling effects is calculated as well. In the absence of spin dephasing, rotations will be limited by the achievable Ω ij / γ ij , with the overall amplitude damping in time t going as tγ ij /2, leading to an infidelity of a π -pulse of order πγ ij /(2Ω ij ). Considering dephasing due to the random, quasi-static nuclear field with characteristic dephasing time , we find for our device parameters that . Therefore, phonon mediated decay does not increase dephasing beyond the hyperfine contribution. Importantly, a quasi-static dephasing contribution (here from the hyperfine field) affects Rabi oscillations less strongly than rapidly fluctuating fields (here from phonons); it permits Rabi oscillations to be observed with periods much longer than [27] , [28] . Table 1 Microwave transitions in the (1,1) spin manifold. Full size table Controllability of the (1,1) manifold can be best achieved by using only the three couplings between the triplet manifold and the singlet, corresponding to the largest Rabi frequencies. With envelope amplitudes of ℏ Ω ≲ 10 μeV, just within the perturbative limits of our theory, Rabi frequencies of order 10 MHz are possible, similar to the frequencies obtained in similar quantum dots for single-spin rotations. Thus, we find that the complete (1,1) subspace is controllable using direct transitions near the S (0,2) crossing, with many rotations possible [3] , [27] , [28] , enabling microwave-induced entangling gates. In addition, our observations suggest new measurement techniques that do not rely on Pauli spin blockade [26] . An example is a measurement that distinguishes parallel from anti-parallel spins while acting non-destructively on the S (1,1)− T 0 (1,1) subspace, which can be achieved by coupling resonantly the T + (1,1) and T − (1,1) states to S (0,2), followed by charge readout. This constitutes a partial Bell measurement and leads to a new method for producing and purifying entangled spin states that enables universal measurement-based quantum computation [29] , [30] , [31] . Sample fabrication 30-nm thick TiAu gates are fabricated on a 90-nm deep (Al 0.3 ,Ga 0.7 )As/GaAs two-dimensional electron gas (2DEG) by means of e-beam lithography. The double-dot axis is aligned along the [110] GaAs crystal direction ( z -direction), which is parallel to the external magnetic field direction ( Fig. 1a ). The 2DEG is Si δ -doped (40 nm away from the hetero-interface), exhibits an electron density of 2.05×10 11 cm −2 and a mobility of 2.06×10 6 cm 2 per Vs at 1 K in the dark. The grounded, 275 nm thick, 2-μm wide and 10-μm long Co μ magnet is evaporated on top of an 80-nm thick dielectric layer, aligned along (magnetic easy axis) and placed ∼ 400 nm away from the closest dot centre. We calculate [32] that, at the double-dot position, the μ magnet adds b 0 ∼ 110 mT to B z and generates a magnetic field gradient of Δ B || ≈ 6 mT per 50 nm and a transverse gradient of Δ B ⊥ ∼ −6 mT per 50 nm at saturation ( B z ≳ 2 T). Measurement The sample is mounted in an Oxford KelvinOx 300 dilution refrigerator at 30 mK. Left and right side gate voltages, V L and V R , are set by low-pass filtered dc lines and ∼ 60 dB attenuated coaxial lines combined with bias-tees with a cutoff frequency of 30 Hz. The pre-amplified current through the quantum-point contact is read out by a lock-in amplifier locked to the 880 Hz on–off modulation of the microwaves. The bias across the double dot is set to 0 μV. Voltage pulses to the left and right side gates are generated with a Sony Textronix AWG520. The microwaves are generated with a HP83650A and combined with the pulses to the right side gate. Microwave bursts and detuning pulses are synchronized to ensure that the microwave excitation is switched off during the detuning pulses that generate the reference signal ( Fig. 1d ). The gates constitute an open-ended termination of the transmission line and, therefore, the microwaves predominantly generate an AC electric field giving rise to purely electric-dipole PAT transitions. The AC magnetic field contribution from the displacement current is negligible at the dot position. The highest contribution is the displacement current from the right side gate to the 2DEG. The separation between them is 90 nm and the shortest distance between the right dot and the displacement current is more than 100 nm. The relevant area of the displacement current is the area of the right side gate closest to the dot, which is roughly 40 nm by 200 nm. At an AC voltage of 1 mV and at the highest frequency of 20 GHz, the displacement current generates an AC magnetic field of less than 2 nT at the right dot, corresponding to a Rabi frequency of 11 Hz. This is three orders of magnitude slower than the spin relaxation time ( Fig. 4 ) and therefore negligible (see also the reasoning in ref. 9 ). Simulation The. Hamiltonian describing the two-spin system near the (1,1)−(0,2) transition is taken to be a five-state system, with four (1,1) spin states and a (0,2) spin singlet [17] in the presence of an external magnetic field B and a magnetic field gradient , which includes both the quasi-static nuclear field and the field from the μ magnet. This is given by , were P 11 is the projector onto the (1,1) subspace, ɛ is the detuning due to the difference in gate potentials from the left and right gates and the tunnel coupling H t = t s (| S (1,1)〉〈 S (0,2)|)+ t SO ( |T + (1,1)〉〈 S (0,2)|)+ t SO ( |T − (1,1)〉〈 S (0,2)|)+h.c with t s the spin-conserving tunnel coupling and t so the spin–orbit coupling set to 5% of t s . To find the signal, we expect theoretically from the experiment, we add a weak, rapidly oscillating term to the Hamiltonian: ɛ → ɛ 0 +Ωcos( vt ). We diagonalize H with Ω=0, then make a rotating frame transformation in which levels are grouped into bands n (defined by a projector P n ) where the states in a band n are much closer in energy than hν , while the energy difference between states in band n and n +1 are within 2/3rds of hν . Each band rotates at a rate nν , and we can then make a rotating wave approximation, keeping terms due to δ that couple adjacent bands, that is, our perturbation in the rotating frame and rotating wave approximation is Next, we add dissipation and dephasing by including relaxation due to coupling of the electron charge to piezoelectric phonons in a two-orbital (Heitler–London-like) model. We thereby neglect deformation phonons as the energy scales examined in the experiment (7–22 GHz) are much smaller than the characteristic frequency scale of a phonon on the length scale of the dot c ph / l do t ∼ 60–120 GHz. To determine the coupling, we take as an ansatz for the electronic wavefunctions the Fock–Darwin states, given by Gaussians, and calculate the coupling after orthogonalizing the states with the perturbation [33] , where f ( k z ) ∼ 1 for the energy scales we are working with. We then use Fermi's golden rule to calculate excitation and relaxation from thermal and spontaneous emission of phonons. Finally, we numerically solve the superoperator for the steady state and compare the expectation value of |S(0,2)〉〈 S (0,2)| with and without the excitation Ω, mimicking the effect of the lock-in detection. Coherent transitions within the (1,1) manifold We conclude with a discussion of the controllability of the (1,1) charge manifold using modulated microwaves on ɛ . To evaluate this, we consider the high-magnetic field, large detuning limit, where where t s is the characteristic tunnelling energy scale. In this limit, we can use a Schrieffer–Wolff transformation for H 0 + V into the (1,1) subspace, where in the basis ( T − (1,1), |↓↑〉, |↑↓〉, T + (1,1), S − (0,2)) with b = gμ B B z , db = gμ B Δ B || . Defining the un-normalized coupling vector , the tunnel coupling is represented by , with We seek S such that exp( λS )( H 0 + λV )exp(− λS ) is block diagonal (has no terms coupling (1,1) to (1,1)) to order λ 2 . Here λ is a perturbation theory parameter that we will take to be unity after the analysis. S is given by solution of P ([ S , H 0 ]+ V ) Q =0, where P projects onto the (1,1) charge space and Q projects onto the (0,2) configuration. It takes the form S =| B 〉〈 S (0,2)|−| S (0,2)〉〈 B| , with Finally, for the (1,1) manifold, we get the effective Hamiltonian to order λ 2 of Within this framework, we can now evaluate the effects to order λ 2 expected from a time-dependent perturbation of the form V 1 =Ω( t )cos( vt )| S (0,2)〉〈 S (0,2)|. We get coupling between (1,1) and (0,2) at order λ , and coupling between (1,1) states at order λ 2 . The charge-changing coupling becomes (taking λ →1): From this expression, we see that microwave transitions are possible through time-dependent driving of ɛ , if | B 〉 has a non-zero matrix element for the desired state. We also see immediately that Raman coupling through | S (0,2)〉 has the same matrix elements as a direct coupling between (1,1) states through the | B 〉〈 B| term. Thus, full controllability of the (1,1) manifold through microwaves can be arrived at by two methods. One is to use stimulated Raman transitions through the | S (0,2)〉 state, the other is to use direct transitions at order λ 2 . Both yield similar coupling strengths so that the stimulated Raman process does not beat the direct process in this case. However, we remark that in the absence of a magnetic field gradient, controllability of the |↑↓〉, |↓↑〉 manifold, without coupling to the | T ± 〉 states, can not be achieved this way, as there is zero coupling through microwaves within this theory to the pure | T 0 〉 state. However, with the magnetic-field gradients in the experiment, controllability is recovered with the constraint that operation pulses cannot be faster than db / ℏ . How to cite this article: Schreiber, L. R. et al . Coupling artificial molecular spin states by photon-assisted tunnelling. Nat. Commun. 2:556 doi: 10.1038/1561 (2011).